Subnanoradian X-ray phase-contrast imaging using a far-field interferometer of nanometric phase gratings Hard X-ray phase-contrast imaging characterizes the electron density distribution in an object without the need for radiation absorption. The power of phase contrast to resolve subtle changes, such as those in soft tissue structures, lies in its ability to detect minute refractive bending of X-rays. Here we report a far-field, two-arm interferometer based on the new nanometric phase gratings, which can detect X-ray refraction with subnanoradian sensitivity, and at the same time overcomes the fundamental limitation of ultra-narrow bandwidths (Δ λ/λ ~10 −4 ) of the current, most sensitive methods based on crystal interferometers. On a 1.5% bandwidth synchrotron source, we demonstrate clear visualization of blood vessels in unstained mouse organs in simple projection views, with over an order-of-magnitude higher phase contrast than current near-field grating interferometers. X-ray imaging commonly relies on the attenuation contrast, in which the visibility of internal structures arises from different levels of radiation absorption. In comparison, phase-contrast imaging, which detects changes in the refractive index from distortions of a wavefront as it propagates through an object, provides an alternative means for distinguishing structures without necessarily depositing significant radiation energy. This idea has stimulated a number of recent innovations [1] . The sensitivity of phase-contrast imaging is characterized by the minimum detectable distortion in the propagating wavefront, which can be quantified by the minimum detectable angle of refractive bending [2] , [3] . To date, the most sensitive methods utilize reflection or diffraction in perfect crystals to either directly detect the refraction of a beam (crystal analyser-based imaging [4] , [5] , [6] ) or to create a coherent interference between two widely separated beams (Bonse–Hart interferometer [7] ). The latter is the most sensitive of all, capable of measuring subnanoradian refraction angles [8] and indeed the absolute phase shift caused by the presence of an object [9] , [10] , [11] . However, the perfect crystals of a Bonse–Hart interferometer select a narrow spectral band (Δ λ / λ ~10 −4 ) that meets the Laue condition of diffraction for a given incident angle [8] , [12] . For common X-ray tubes, almost all of the flux would be lost, leading to long exposure times. Alternatively, methods based on free-space propagation of a transversely coherent wavefront are well suited for polychromatic sources [13] , [14] . A coherent wavefront passing through a grating also produces a self-image of the grating in the near field (the Talbot effect), which allows phase-contrast imaging with polychromatic sources [15] , [16] . The requirement for lateral coherence is further relaxed in the Talbot–Lau grating interferometers [17] , which includes an additional absorption grating in front of the source. Furthermore, the refractive bending of X-rays can be directly observed by the movement of the Fresnel diffraction fringes of a sharp edge under polychromatic illumination [18] , [19] . However, for systems of similar lengths, the perfect crystal interferometers achieve the highest sensitivity [2] , [8] , [20] . With the near-field Talbot or Talbot–Lau interferometers, the idea of improving sensitivity by reducing the grating period also faces both inherent and practical limitations. As the Talbot self-imaging effect is inherently a near-field phenomenon, where the Talbot distance decreases quadratically with the grating period, a wave propagation distance of 1.0 m becomes ~700 times the Talbot distance for a 200-nm grating period and X-ray photon energy of 22.5 keV. Thus, small grating periods put the system in the far-field range, where the Talbot effect diminishes [21] , [22] . Talbot interferometers also utilize absorption gratings to form moiré fringes, which at submicron periods are structures of extreme aspect ratios, posing remarkable challenges for fabrication [23] , [24] . Considering the above limitations, a desirable candidate for further raising phase-contrast sensitivity would be a far-field interferometer, consisting only of phase gratings and be compatible with polychromatic and divergent sources. Here we describe the grating Bonse–Hart (GBH) interferometer that meets these requirements. Polychromatic interferometry is exemplified by the versatile Mach–Zehnder interferometer [25] , in which two symmetric beams of equal path lengths produce achromatic interference fringes. The X-ray Bonse–Hart interferometer is such an interferometer that uses monolithic crystals in place of mirrors [7] . Here, by replacing the crystals with nanometric phase gratings, we remove the strict wavelength filtering of the crystals and arrive at a GBH interferometer. The simplest configuration of the GBH interferometer consists of three identical phase gratings of period P arranged in equally spaced parallel planes ( Fig. 1a ). The X-ray detector is positioned down beam from the third grating at the same spacing. 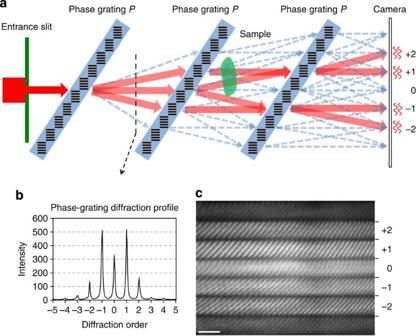Figure 1:TheP-P-Pconfiguration of the GBH interferometer. (a) The simplest GBH configuration consists of three identical phase-shift gratings. The experimental system used multilayer gratings of 200 nm period and 1.4πphase shift. The diffraction profile of a grating is plotted inb. By using an entrance slit, the network of diffraction pathways are separated into bands on the image plane. Two pairs of symmetric pathways give rise to four pairs of mutually coherent beams (solid red arrows). They produce interference fringes in the ±1 and ±2 bands. Some of the other pathways (dotted arrows) also fall into these bands and contribute a background intensity. An intensity image is shown inc. Scale bar, 200 μm. The average fringe visibility in the +1 band, defined as (Imax−Imin)/(2Iaverage), was 12%. The 2P-P-2P configuration withπphase-shift gratings was shown to attain near-ideal fringe visibility in a visible light analogue (Supplementary Fig. S5). Figure 1: The P - P - P configuration of the GBH interferometer. ( a ) The simplest GBH configuration consists of three identical phase-shift gratings. The experimental system used multilayer gratings of 200 nm period and 1.4 π phase shift. The diffraction profile of a grating is plotted in b . By using an entrance slit, the network of diffraction pathways are separated into bands on the image plane. Two pairs of symmetric pathways give rise to four pairs of mutually coherent beams (solid red arrows). They produce interference fringes in the ±1 and ±2 bands. Some of the other pathways (dotted arrows) also fall into these bands and contribute a background intensity. An intensity image is shown in c . Scale bar, 200 μm. The average fringe visibility in the +1 band, defined as ( I max − I min )/(2 I average ), was 12%. The 2P-P-2P configuration with π phase-shift gratings was shown to attain near-ideal fringe visibility in a visible light analogue ( Supplementary Fig. S5 ). Full size image In general, each grating produces several diffraction orders, including the zeroth order ( Fig. 1b ). Sequential diffractions by the gratings produce a network of light paths ( Fig. 1a ). These can be labelled by the diffraction orders of the gratings as ( j , k , l ). Because of the symmetry of the grating arrangement, there are pairs of symmetric pathways of equal path lengths, which converge at the third grating and copropagate in parallel to the detector ( Fig. 1a ). An example is the (+1, −1, 0) and (0, +1, −1) paths. The pair of beams sum either constructively or destructively on the image plane, depending on the phase difference between them. A key characteristic of the system is that the phase difference between a symmetric pair of pathways is determined by the relative positions of the grating lines, and independent of both the wavelength and the incident angle [26] . Thus, the fringe patterns from different wavelengths and incident angles are aligned in phase to each other (a more detailed discussion is provided with Supplementary Fig. S1 ). This feature enables the interferometer to use broadband and extended sources. However, phase-shift gratings are not expected to produce coherent interference effects without a highly collimated incident beam. As phase gratings by definition do not appreciably modulate the intensity of a wavefront, they do not improve the transverse coherence of the incident beam. Another way to state the problem is that when all diffraction pathways overlap on the image plane, the sum at any location approaches a constant due to energy conservation, resulting in a flat, featureless field. This problem was demonstrated in a visible light analogue using a broadband white light source [26] . The solution was also found in the visible light analogue, that is, combining high-density gratings of sufficiently large diffraction angles with slits along the beam to separate the diffraction pathways on the image plane. In the simplest embodiment, horizontal entrance slits are used to limit the height of the incident beam, which result in vertically separated groups of diffraction pathways on the image plane ( Fig. 1a ). Here we implement the above concept on a synchrotron source of 1.5% spectral bandwidth (2-BM-B, APS, Argonne National Laboratory, IL, USA) and perform a number of phase-contrast imaging experiments. We find the X-ray GBH interferometer to behave as a classic two-arm interferometer. It achieves high sensitivity towards subtle phase variations of the X-ray wavefront at moderate radiation doses. Absolute phase-shift imaging Samples that are smaller than the 160-μm height of the entrance slit can fit into one of the two interfering beams, whereas the other beam serves as a phase reference. This configuration measures the absolute phase shift incurred by the sample. For example, the absolute phase shifts in polystyrene beads of 100 μm diameters were compared with theoretical profiles calculated from the refractive index of polystyrene at 22.5 keV ( http://www.nist.gov/pml/data/ffast/index.cfm ; Fig. 2 ). For a statistical comparison, the maximum phase shift at the centre of the beads (after phase unwrapping) was measured to be 5.19±0.31 radians ( n =7), corresponding to a material refractive index of 1−(4.56±0.27) × 10 −7 . This was in agreement with the reference value of (1−4.68 × 10 −7 ) for polystyrene. 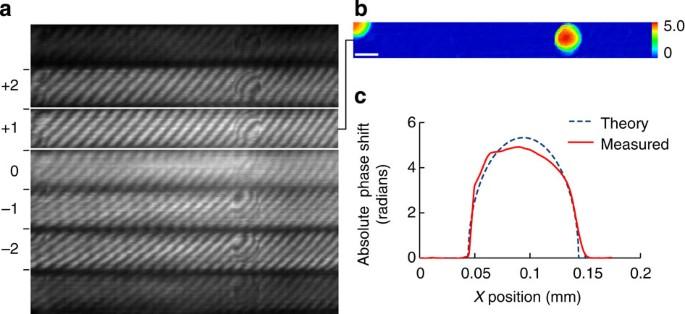Figure 2: Absolute phase-shift measurements of polystyrene beads. (a) Polystyrene beads of 100 μm diameters can fit into one of the two interfering beams of the GBH interferometer. Phase shifts incurred by the beads alter the positions of the interference fringes in the separate diffraction bands of the image. (b) The +1 band was used to retrieve an absolute phase-shift image. Scale bar, 100 μm. (c) The measured phase-shift profile across a bead is plotted with the theoretical profile. Theoretical values can be calculated from the refractive index of polystyrene at 22.5 keV, assuming a perfect spherical shape for the beads. Statistical results from these comparisons are given in the text. Figure 2: Absolute phase-shift measurements of polystyrene beads. ( a ) Polystyrene beads of 100 μm diameters can fit into one of the two interfering beams of the GBH interferometer. Phase shifts incurred by the beads alter the positions of the interference fringes in the separate diffraction bands of the image. ( b ) The +1 band was used to retrieve an absolute phase-shift image. Scale bar, 100 μm. ( c ) The measured phase-shift profile across a bead is plotted with the theoretical profile. Theoretical values can be calculated from the refractive index of polystyrene at 22.5 keV, assuming a perfect spherical shape for the beads. Statistical results from these comparisons are given in the text. Full size image Phase-difference imaging and phase unwrapping In larger samples, both of the interfering beams propagate in the sample, resulting in a phase-difference image between the locations of the two beams (see Methods section for a detailed description). Insect samples offer many fine features with sharp changes in the refractive index, for example, between the solid skeletal structures, fluid tissue and air compartments. They are often used in X-ray phase-contrast experiments [27] , [28] , [29] , [30] . With the GBH interferometer, a fruit fly was imaged in a vertical tile of 19 fields of view. Owing to the sensitivity of the instrument, the measured phase-difference values reached several times of π in the torso of the fly and resulted in multiple fold of phase wrapping ( Fig. 3a ). Phase unwrapping using a combination of line-cut [31] , [32] , [33] and signal-to-noise ratio-weighted [34] algorithms proved to be able to remove the phase wraps, except in some spots of dense skeletal parts that contained abrupt and large jumps in phase, which caused ambiguity in the assignment of phase [35] ( Fig. 3b ). In soft tissue samples discussed below, the phase maps are sufficiently smooth to avoid such ambiguities. 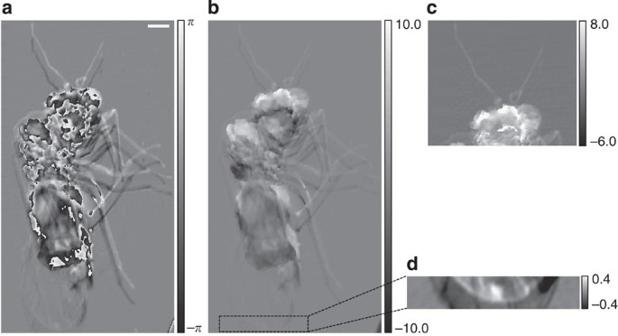Figure 3: Phase-contrast images of a fruit fly. (a) The GBH interferometer retrieves a phase-difference image of the fruit fly, which contains phase wraps in the body. It is the sum of two phase-shift images of opposite signs, with a vertical offset of 140 μm. Scale bar, 200 μm. (b) The unwrapped phase-difference image. (c) By a shift-and-sum algorithm, an absolute phase-shift image of the head portion of the fly was retrieved. The wingtip area outlined with a dotted rectangle inbis magnified indand shown in a smaller grey scale. From the phase-shift values in this area, the thickness of the wing membrane could be estimated. Figure 3: Phase-contrast images of a fruit fly. ( a ) The GBH interferometer retrieves a phase-difference image of the fruit fly, which contains phase wraps in the body. It is the sum of two phase-shift images of opposite signs, with a vertical offset of 140 μm. Scale bar, 200 μm. ( b ) The unwrapped phase-difference image. ( c ) By a shift-and-sum algorithm, an absolute phase-shift image of the head portion of the fly was retrieved. The wingtip area outlined with a dotted rectangle in b is magnified in d and shown in a smaller grey scale. From the phase-shift values in this area, the thickness of the wing membrane could be estimated. Full size image The detector resolution was sufficient to clearly resolve the two overlapping phase images of opposite signs with a vertical offset of 140 μm between them (the origin of the twin images is explained in the Methods section). A discrete shift-and-sum algorithm to retrieve a single phase image has been formulated in X-ray phase-contrast microscopy [36] , provided that there are sufficient empty areas above and below the sample. A slightly modified version that requires an empty margin at one end of the image proved effective in retrieving the phase shift in areas where phase wrapping was fully resolved ( Fig. 3c ). As a demonstration of the inherent sensitivity of phase contrast relative to attenuation contrast, the absolute phase shifts in the distal end of the wing membrane ( Fig. 3d ) were found to range between 0.05 and 0.15 radians. On the basis of the refractive index of chitin [37] ( http://www.nist.gov/pml/data/ffast/index.cfm ), the primary constituent of insect wings, the thickness of the wing membrane was estimated to be between 0.6 and 1.8 μm in this area. The corresponding intensity attenuation of (0.5~1.5) × 10 −4 was undetectable by our 12-bit camera. Soft tissue imaging compared with a Talbot interferometer In soft tissue samples without air pockets, the measured phase difference was found to vary smoothly when compared with the insect body. A freshly excised kidney specimen from a 3-week-old male mouse (C57BL/6 wild type) was first fixed in 10% buffered formalin, then immersed in water-filled vials to remove any air/tissue interfaces. We compared the level of phase contrast of the GBH interferometer with a near-field Talbot interferometer, which was installed on the same synchrotron source. The Talbot interferometer was constructed with a 4.80-μm period π /2 phase grating and an absorption grating of the same period (Microworks GmbH), with the same intergrating distance (the third-order fractional Talbot distance of 0.63 m) and photon counts per pixel as that of the GBH instrument. The absorption grating provided moiré fringes of 32% visibility. An air bubble was introduced into the sample vial of the Talbot interferometer to produce a high phase-contrast signal as a way to verify its correct function. Blood vessels in the kidney were highlighted by their phase contrast in a single projection image from the GBH interferometer ( Fig. 4a ). Their sizes were between 100 and 300 μm. Their identities were confirmed by a comparison with a three-dimensional magnetic resonance imaging scan ( Fig. 4d ). In a blood vessel of ~200 μm diameter, the phase-difference signal from the GBH was about 15 times the differential phase signal from the Talbot interferometer ( Fig. 4c ), which is consistent with the estimated ratio from the derivative approximation of the GBH phase-difference signal (equation (3)). The differential phase image from the Talbot interferometer ( Fig. 4b ) reveals high phase contrast at the air–water interface of the bubble [17] , [38] , but limited visibility of the blood vessels. 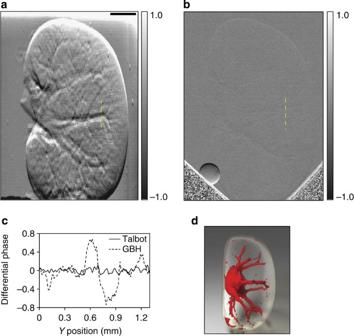Figure 4: Phase-contrast images of a water-immersed mouse kidney specimen. (a) A phase difference image acquired with the GBH interferometer of a mouse kidney specimen held in a water-filled vial. Scale bar, 1.0 mm. (b) The differential phase image acquired with the Talbot interferometer of the same specimen, held in a separate water-filled vial where an air bubble was introduced to provide strong phase contrast at the water–air interface. (c) Line profiles along the dashed lines inaandbare plotted for comparison. (d) A volume-rendered view of a three-dimensional magnetic resonance imaging (MRI) data of the specimen shows the disposition of the blood vessels in the kidney. The MRI data helped to identify the features seen in the X-ray phase-contrast images as blood vessels. Figure 4: Phase-contrast images of a water-immersed mouse kidney specimen. ( a ) A phase difference image acquired with the GBH interferometer of a mouse kidney specimen held in a water-filled vial. Scale bar, 1.0 mm. ( b ) The differential phase image acquired with the Talbot interferometer of the same specimen, held in a separate water-filled vial where an air bubble was introduced to provide strong phase contrast at the water–air interface. ( c ) Line profiles along the dashed lines in a and b are plotted for comparison. ( d ) A volume-rendered view of a three-dimensional magnetic resonance imaging (MRI) data of the specimen shows the disposition of the blood vessels in the kidney. The MRI data helped to identify the features seen in the X-ray phase-contrast images as blood vessels. Full size image In previous Talbot and Talbot–Lau interferometer studies of similar resolutions, vascular structures have been visualized in computed tomography scans combining a large number of projection views [39] , [40] , [41] , [42] , resulting in dose levels that are several orders of magnitude above the current study. However, we have not found such examples in single projections in the literature [40] , [43] , [44] , [45] . The examples of unstained vascular imaging in projection radiography have so far been provided by the extremely sensitive crystal Bonse–Hart interferometer [46] , [47] . The results we obtained from the Talbot and GBH interferometers are consistent with these prior findings. To retrieve the phase shift from the phase-difference image, we used the derivative approximation represented by equation (4) in the Methods section. The phase shift could then be obtained by integration with an appropriate scaling factor. A high-pass spatial filter with a threshold of 0.5 mm was applied in the vertical direction to remove noise streaks that arise in the integration process [48] . This procedure was applied to both the GBH and Talbot interferometer data. The results are summarized in Fig. 5 . The GBH phase-shift image yields a projection view of the blood vessels. The Talbot phase-shift image shows strong phase shifts in the air bubble and reduced visibility of the blood vessels relative to the GBH data. 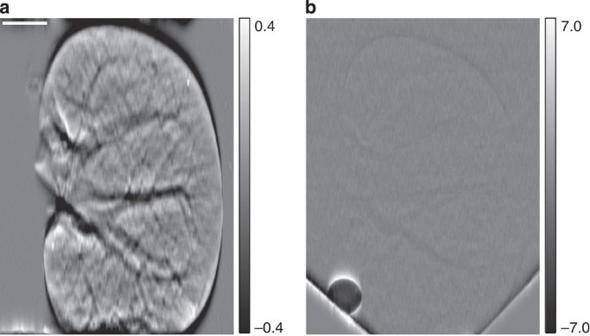Figure 5: Integrated phase-shift images of the mouse kidney specimen. (a) An image of the phase shift in the mouse kidney from the GBH interferometer provides a projection view of the blood vessels. By approximating the phase-difference data as a derivative measurement of the phase shift, it is integrated in the vertical direction into a phase-shift image, then high-pass filtered to remove vertical streak artifacts. Scale bar, 1.0 mm. (b) The same integration method was used with the differential phase data from the Talbot interferometer. It provided a phase-shift image of the same specimen in a different water-filled vial that contained an air bubble. The bubble causes a strong phase shift relative to the surrounding water. Several blood vessels are faintly visible against the background noise. Figure 5: Integrated phase-shift images of the mouse kidney specimen. ( a ) An image of the phase shift in the mouse kidney from the GBH interferometer provides a projection view of the blood vessels. By approximating the phase-difference data as a derivative measurement of the phase shift, it is integrated in the vertical direction into a phase-shift image, then high-pass filtered to remove vertical streak artifacts. Scale bar, 1.0 mm. ( b ) The same integration method was used with the differential phase data from the Talbot interferometer. It provided a phase-shift image of the same specimen in a different water-filled vial that contained an air bubble. The bubble causes a strong phase shift relative to the surrounding water. Several blood vessels are faintly visible against the background noise. Full size image Refraction angle sensitivity The sensitivity of the GBH interferometer was quantified as the noise level in the measured refraction angle of an X-ray beam [2] , [3] , [8] . This is given by (Δ ϕ /2 π )( P / D ), where Δ ϕ is the noise level of the phase-difference image, P is the grating period and D is the distance between the sample and the third grating. The phase-noise level, determined as the s.d. of the pixel values in empty background areas, was (1.19±0.25) × 10 −2 radians from measurements in eight different background locations in the data shown in Fig. 3 . Correspondingly, the noise level in the X-ray refraction angle was 0.63±0.13 nrad. Radiation dose and spatial resolution The above sensitivity was obtained at a 23-Gy skin dose on the sample, which was estimated from the total exposure time of 30 s over the phase-stepping process and the photon flux of the synchrotron beamline (8.7 × 10 10 ph mm −2 s), taking into account the attenuation in the substrates of the two gratings before the sample and the beam spreading effects of grating diffraction. To project the dose value to typical radiography exams, we need to consider the scaling with the pixel size and the detector quantum efficiency (DQE). Replacing the current detector of 1.6 μm pixel size and DQE of 0.21 with a digital flat-panel detector of 50 μm pixel size and DQE of 0.3, the estimated skin dose is given by 23 Gy·(1.6 μm per 50 μm) 2 ·(0.21/0.3)=17 mGy. The estimated mean glandular absorption dose is given by 0.155·(skin dose)=2.6 mGy for 25 keV radiation through a 4.5-cm tissue layer [49] . This level of radiation is comparable to the 3 mGy limit for a mammogram established by the American College of Radiology [50] . Interestingly, a closer inspection revealed that the phase noise was dominated by structured patterns in the background (detailed information is provided with Supplementary Fig. S2a ). They are likely the result of imperfections in the gratings ( Supplementary Fig. S2b ) and the temporal fluctuation of the intensity pattern of the synchrotron source ( Supplementary Fig. S2c ). This indicates that the current limiting factor for sensitivity is systematic errors instead of the radiation dose. The spatial resolution of the GBH interferometer is dependent on whether to interpret the measured data as a discrete phase-difference measurement (equation (3) in the Methods section) or to apply the derivative approximation (equation (4) in the Methods section). The first choice may be better suited for microscopy applications where discrete algorithms will be used to separate the twin phase images. For macroscopic imaging, the derivative approximation is more robust, particularly when using X-ray tube sources of broad spectral widths. Specifically, the separation d between the two interfering beams in the sample will span a range, which is given by D (Δ λ / P ), where Δ λ is the bandwidth of the source. A trade-off of the derivative approximation is that it ‘blurs’ the differential phase data by the average beam separation d . For a compact imaging system using an X-ray tube centred at 35 keV, with a grating period of 200 nm and an intergrating distance of 0.4 m, the beam separation reaches 70 μm. As the pixel elements in the typical flat-panel detectors range between 50 and 500 μm, the beam separation is not expected to substantially have an impact on the image resolution when using these detectors. The question of how the detector pixel size influences the visibility of phase objects was addressed with numerical simulations. We simulated the phase-difference signal from cylinders of water buried in typical soft tissue (ICRU 4-component tissue, http://physics.nist.gov/cgi-bin/Star/compos.pl?matno=262 ) for cylinder diameters of 50, 100, 200 and 500 μm, and pixel sizes of 1.6 and 50 μm. The cylinders were placed perpendicular to the X-ray beam and parallel to the grating lines. The simulation modelled the measured phase-difference value of a finite pixel as the average of all points in the pixel. Specifically, the phase difference signal φ ( r ) at a point r on the detector plane is expressed by equation (3) in the Methods section. The phase-difference signal φ ′( R ) measured by a finite pixel at location R was given by The simulated instrument parameters were 35 keV photon energy, 40 cm intergrating distance and 200 nm grating period. The simulation results are graphed in Fig. 6 . For the 200 and 500 μm diameter cylinders, the two pixel sizes provided similar phase-difference profiles or similar visibility of the cylinders. For the 100-μm and particularly the 50-μm cylinder, the detected phase contrast from the 50-μm pixel size is less than that of the 1.6-μm pixel size. The results show that the visibility of an object is largely independent of the pixel size until the pixel size grows to approach the size of the object, at which point the visibility decreases. This is in addition to the general sampling rule that an object needs to span at least several pixels to be resolved in a discrete image. 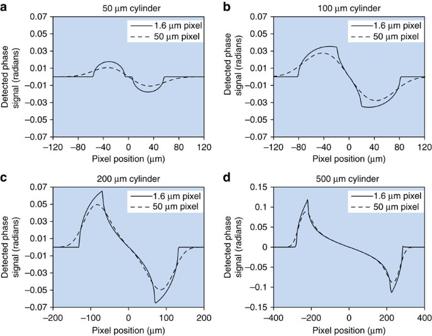Figure 6:Simulated phase-differenceprofiles. The simulated samples contain water cylinders with various diameters immersed in typical soft tissue (NIST ICRU four-component tissue model). The detected phase-difference signal profiles across the diameter of the cylinders are graphed as functions of the pixel position. The cylinder diameters ranged between 50 and 500 μm (a–d). Two detector pixel sizes of 1.6 and 50 μm were simulated. The graphs show that the detected phase contrast is similar between the two pixel sizes in the 200 and 500 μm cylinders, whereas in the smallest 50 μm cylinder the phase contrast seen with the 50 μm pixel size is substantially lower than that from the 1.6 μm pixel size. Figure 6: Simulated phase-difference profiles. The simulated samples contain water cylinders with various diameters immersed in typical soft tissue (NIST ICRU four-component tissue model). The detected phase-difference signal profiles across the diameter of the cylinders are graphed as functions of the pixel position. The cylinder diameters ranged between 50 and 500 μm ( a – d ). Two detector pixel sizes of 1.6 and 50 μm were simulated. The graphs show that the detected phase contrast is similar between the two pixel sizes in the 200 and 500 μm cylinders, whereas in the smallest 50 μm cylinder the phase contrast seen with the 50 μm pixel size is substantially lower than that from the 1.6 μm pixel size. Full size image We showed experimentally that an X-ray far-field interferometer consisting of phase gratings functions similarly to a crystal Bonse–Hart interferometer, but at 100 times the bandwidth, with no inherent limitations regarding the use of broadband compact sources. The 0.63-nrad refraction sensitivity is an order-of-magnitude improvement over other systems of similar sizes, including grating Talbot interferometers using synchrotron sources [39] and free-electron laser [3] (10–15 nrad sensitivity), and direct refraction imaging with monochromatic crystal analysers at synchrotron sources [6] , [20] (10–40 nrad sensitivity). It is also a factor of three improvement over refraction measurements by the edge illumination method over 10–15 m distances [19] (1.9 nrad). Although the sensitivity still falls somewhat short of the crystal Bonse–Hart interferometer [8] (0.1 nrad), its broader bandwidth should allow shorter exposure times with compact sources. In the current implementation, the phase noise arises from the imperfections in the first-generation nanometric gratings and from beam pattern fluctuations, leaving room for further improvements in sensitivity and dose reduction. When compared with near-field grating interferometers, the amplified phase contrast is accompanied by more frequent phase wrapping. Phase unwrapping is principally constrained by the need for sufficient smoothness of the underlying phase variation. Specifically, the phase change within a pixel should be less than π to avoid ambiguity in the assignment of phase [35] . Therefore, the resolution of the imaging system should match the ‘steepness’ of the phase variation. For example, in a compact imaging system centred at 35 keV with a pixel size of 50 μm, the wavefront accumulates a π phase shift in a soft tissue layer of 95 μm. This is the effective limit of the change of tissue thickness within a pixel. The main limitation of the GBH interferometer is the small vertical field of view imposed by the slits. The slits are essential for separating the diffraction orders of the phase gratings in a far-field interferometer. A future solution to this problem is to employ arrays of parallel slits to expand the vertical field of view. The current width of the slit was 160 μm, and typical compact systems will have slits of tens of microns and wider ( Supplementary Fig. S3 ). The fabrication of such slit arrays would be less challenging than the current absorption gratings for Talbot–Lau interferometers having periods of several microns. These are commercially available from several sources (for example, Microworks GmbH and Creative MicroTech Inc.) in overall sizes up to 10 cm, slit widths down to 2.4 μm and X-ray photon energies up to 50 keV. The commercial products are generally periodic polymer structures with gold-filled trenches, fabricated with X-ray or ultraviolet lithography followed by electroplating. Given the relatively large widths of the slits, the alignment of the slit arrays could be performed using the X-ray beam and the detector themselves as the tools. In the absence of the nanometric gratings, X-ray transmission through the slits follows simple projections (geometric optics). Thus, an alignment procedure would start with two slit arrays in the X-ray beam. Any slight rotation between the two arrays will result in broad moiré fringes on the detector. By adjusting the angle and position of one array to remove the moiré pattern and maximize the transmitted intensity, the two arrays would be aligned. Next, additional slit arrays could be added one-by-one and aligned using the same procedure. Once the slit arrays are aligned, the phase gratings can then be put in place. To address the question about alignment stability of such slits in a compact system, we look to a recent study by Tapfer et al. [51] on the stability of a Talbot–Lau interferometer mounted on a gantry of about 0.9 m length, with gratings of 3.4–10.0 μm periods. The study found that the most significant thermal drift was in the source grating, ranging from −1 to 5 μm in a period of 4 h. It was attributed to direct thermal conduction from the X-ray tube to the mounting of the grating. Although this level of drift is small compared with our slit dimensions, the study points to the value of reducing thermal contact between the X-ray tube and the rest of the system to reduce thermal drifts. The system is much more sensitive to changes in the alignment of the nanometric phase gratings. Experimentally measured drifts and effect ways to deal with them are described in the Methods section. In general, if the mechanical drift over the exposure time of a single image is small relative to the grating period, it will not degrade individual images and can be effectively dealt with in post processing. For example, the drift observed by Tapfer et al. [51] had a maximum rate of 4 μm h −1 , or 7 nm over a 6-s exposure, which is small relative to a grating period of 200 nm. However, rapid vibrations that may be present in a continuously rotating computed tomography system are more challenging to remove and may require higher imaging frame rates. A more generalized version of the idea of slit arrays is the use of composite gratings that combine dense phase modulation with long-scale amplitude modulation. The optimal design and combination of such composite gratings in far-field interferometers is a topic for further theoretical and numerical studies. Implementation of the GBH interferometer The phase gratings in this implementation were of 200 nm periods and provided an estimated phase modulation of 1.4 π . The diffraction pattern of an individual grating showed that most of the incident flux was diffracted into the five diffraction orders ranging from −2 to +2 ( Fig. 1b ). Among the network of diffraction pathways, there were four pairs of mutually coherent beams that formed four distinct bands on the image plane ( Fig. 1a ). These are labelled ±1 and ±2 ( Fig. 1a,c ). A slight misalignment of the gratings created a gentle slope in the phase difference between each pair of beams, leading to broad interference fringes in these bands ( Fig. 1c ). A number of other incoherent pathways also fell on the bands ( Fig. 1a ), which decreased the overall fringe visibility to 12% (detailed information is provided with Supplementary Fig. S4 ). We found previously that it is possible to avoid such mixing by combining π phase-shift gratings of two different periods in a 2 P - P -2 P configuration. This was demonstrated in ref. 26 to obtain near-ideal fringe visibility in the visible light analogue with a white light source. The details are summarized with Supplementary Fig. S5 . Although the phase shift of a grating is wavelength dependent (for a tungsten/silicon π shift grating at 22.5 keV, it varies from 0.82 π to 1.28 π over the range of 17.5–27.5 keV), numerical simulations showed that the influence on the efficiency of the interferometer was weak (fringe visibility decreases by <30%) over a bandwidth of 45% (ref. 26 ). Here in this first iteration of the X-ray interferometer, the simple P - P - P configuration of Fig. 1a was implemented. Although the fringe visibility was below the 32% level of a Talbot interferometer of the same intergrating distance (detailed in the following sections), the amplified phase contrast of the GBH interferometer yielded substantially higher overall sensitivity, which is discussed below. The intergrating spacing was 0.65 m. The APS 2-BM-B beamline was a bending-magnet synchrotron beam centred at 22.5 keV. The spectral width of the beam was set by the multilayer mirror of the beamline to 1.5%. Thus, the interferometer operated at a bandwidth that was two orders of magnitude above that of a crystal Bonse–Hart interferometer. The entrance slit limited the height of the incident beam to 160 μm ( Fig. 1a ) and also determined the vertical field of view. A solution to this limitation in the form of slit arrays is discussed at the end of the paper. In general, the height of an individual slit h and the angular divergence Δ of the incident beam should allow separation between adjacent diffraction orders on the image plane. Mathematically, the condition can be expressed as h / L +2Δ< λ / P , with a grating period P and intergrating distance L . In the hard X-ray energy range of 10–100 keV, submicron grating periods become necessary to allow slits of tens of microns or larger sizes (see Supplementary Fig. S3 for numerical plots of the slit height and beam divergence as functions of the grating period). A grating design of multilayer arrays was created to realize the 200-nm period for X-rays in the 17.5–40 keV range. The fabrication and metrology of the gratings are described in some detail in ref. 52 . The design extends the idea of Kim et al. [53] of using a multilayer stack as a transmission grating. To overcome the limited height of the multilayer deposition (tens of microns), we deposited alternating layers of tungsten and silicon onto a stair-like substrate. The effective vertical height of the grating becomes the height of the multilayer stack multiplied by the number of steps. In the first iteration of such gratings, the size of the usable area of a grating was a few millimetres. The grating period was the thickness of a tungsten–silicon bilayer. The horizontal field of view of the GBH instrument was set by the camera to 3.2 mm. The X-ray detector was a 2,048 × 2,048 pixel Coolsnap K4 camera equipped with a × 5 objective lens focusing on a scintillator crystal. The pixel size was 1.6 × 1.6 μm 2 after accounting for the magnification of the objective. The exposure time of each image was 5 s, which gave an average X-ray photon count of 4.0 × 10 4 photons per scintillator area covered by a camera pixel. The raw images were convolved with a square box of 6 × 6 pixels to remove modulations from grating substrate structures, resulting in an effective image resolution of 9.6 × 9.6 μm 2 . Phase-contrast images at full detector resolution were retrieved by the phase-stepping process [9] , [16] , [28] , which consisted of a set of six images taken while the centre grating was moved vertically in 40 nm steps. One of the four bands on the image plane was selected for processing (usually the +1 or −1 band for its slightly higher intensity). The sensitivity of the instrument meant that thermal drift and other mechanical instabilities could cause substantial variation in the phase steps. Experimental data showed that in a period of 15 min, the interference fringes drifted by 0.6 periods, corresponding to a grating alignment drift of 0.12 μm ( Fig. 7 ). An adaptive algorithm was created to process data of arbitrary and spatially varying phase steps without assuming a priori knowledge. We retrospectively determine the phase increments by a Fourier analysis of the interference fringes [54] , [55] . The results were fed into a pixel-wise least-squares fitting process to retrieve the phase images. A reference data set was also acquired without any sample to correct for background instrumental phase variations. 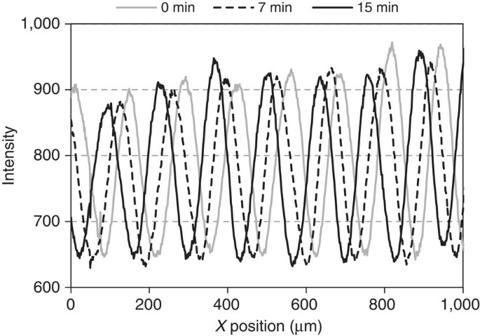Figure 7:The stability of interferencefringe pattern. The drift of the interference fringe pattern is introduced by the mechanical drift of the grating alignment. Intensity line profiles over the same location in a series of reference images taken over a period of 15 min show a drift of the fringe pattern. The three profiles taken at 0, 7 and 15 min are graphed. The amount of drift was 60% of a fringe period over 15 min. It indicates that the alignment of the phase gratings shifted by 0.6 of the grating period in this duration, or 0.12 μm. Figure 7: The stability of interference fringe pattern. The drift of the interference fringe pattern is introduced by the mechanical drift of the grating alignment. Intensity line profiles over the same location in a series of reference images taken over a period of 15 min show a drift of the fringe pattern. The three profiles taken at 0, 7 and 15 min are graphed. The amount of drift was 60% of a fringe period over 15 min. It indicates that the alignment of the phase gratings shifted by 0.6 of the grating period in this duration, or 0.12 μm. Full size image For future compact imaging devices with cone-beam sources, an electronic phase-stepping method was also developed, which realizes phase stepping without moving parts and thereby allows all components to be rigidly mounted for better stability [56] . The method is based on the idea that in the presence of interference fringes, phase-stepping is equivalent to a relative movement between the fringes and the projection image of the sample. By electromagnetically shifting the focal spot of the cone beam, the projection image is displaced in the opposite direction relative to a static fringe pattern, or both are displaced but by different amounts. The images are then digitally shifted to realign the projections, resulting in the appearance of moving fringes over a static projection. This effectively synthesizes the phase-stepping process. In practice, a solenoid coil is attached to the X-ray tube housing. The coil is energized with a digitally controlled current source, which produces a magnetic field in the tube. The field deflects the electron beam in the tube, which shifts its impact point on the anode target where the X-rays are emitted. Phase-contrast imaging experiments The phase signal measured by the GBH interferometer is the difference between the phase shifts of the two mutually coherent beams, which propagate through separate locations in the sample ( Fig. 1a ). The two locations are offset vertically by the distance where D is the propagation distance from the sample to the third grating and P is the grating period. When the image resolution is finer than the distance d , we acquire a discrete phase-difference image with the appearance of twin images of opposite signs as where ϕ ( r ) is the phase shift of the wavefront incurred by the sample. If the image resolution is comparable or larger than the vertical separation d , the twin images are no longer resolved. The phase-difference image is approximated in terms of the derivative of the phase shift: This derivative approximation has the same form as the differential phase signal measured with near-field Talbot and Talbot–Lau interferometers [16] , [17] . The difference is in the distance d , which is an ‘amplification factor’ of the phase contrast. It scales inversely with the grating period (equation (2)). With the derivative approximation, we can estimate the relative levels of differential phase signals between the far- and near-field interferometers. For example, comparing a Talbot interferometer of 4.8 μm grating period and a 200-nm period GBH interferometer of the same wave propagation distance, the differential phase signal should increase by about 24-fold if the underlying gradient of refractive index extends over a distance that is larger than the beam separation d of the GBH interferometer. This was born out by experimental data described below. The derivative approximation also permits integral-based methods to retrieve phase-shift images [48] . At the trade-off of resolution, we found it to be more robust than discrete algorithms, which are well suited for microscopic imaging and directly operate on the phase-difference images [36] . In this study, both the phase difference and differential phase treatments are demonstrated with samples of various scales. How to cite this article: Wen, H. et al. Subnanoradian X-ray phase-contrast imaging using a far-field interferometer of nanometric phase gratings. Nat. Commun. 4:2659 doi: 10.1038/ncomms3659 (2013).